Detection and differential diagnosis of colon cancer by a cumulative analysis of promoter methylation Alterations in the methylation of promoters of cancer-related genes are promising biomarkers for the early detection of disease. Compared with single methylation alteration, assessing combined methylation alterations can provide higher association with specific cancer. Here we use cationic conjugated polymer-based fluorescence resonance energy transfer to quantitatively analyse DNA methylation levels of seven colon cancer-related genes in a Chinese population. Through a stepwise discriminant analysis and cumulative detection of methylation alterations, we acquire high accuracy and sensitivity for colon cancer detection (86.3 and 86.7%) and for differential diagnosis (97.5 and 94%). Moreover, we identify a correlation between the CpG island methylator phenotype and clinically important parameters in patients with colon cancer. The cumulative analysis of promoter methylation alterations by the cationic conjugated polymer-based fluorescence resonance energy transfer may be useful for the screening and differential diagnosis of patients with colon cancer, and for performing clinical correlation analyses. Mortality from colorectal cancer has been on the rise all over the world. Early treatment seems to be a key factor in reducing the death rate of this disease. To help physicians facilitate further examination and initiate treatment, gene-related changes, such as mutation, modification and rearrangements, have been extensively investigated [1] , [2] , [3] , [4] , [5] , [6] . Among them, changes in DNA methylation are some of the most common molecular alterations in human colorectal cancer [1] , [2] , [3] , [5] . As the methylation of gene promoter is responsible for silencing of several critical inhibitory cancer genes, the alterations of methylation levels and patterns can lead to abnormal growth of the cell [1] , [2] , [5] . In particular, promoters of specific genes are aberrantly methylated at different stages of tumour development, that is, different clinical stages and histological types of tumours exhibit a specific methylation phenotype, which could assist physicians to accurately classify tumour stages, assess prognosis and optimize treatments [5] . In recent years, DNA methylation has been increasingly utilized as a marker for cancer detection and differential diagnosis. A number of promoter methylations in cancer-related genes possess well-documented prognostic and predictive value [5] , [7] , [8] . For instance, vimentin ( VIM ) gene methylation, a methylation biomarker has been used in a commercial DNA test (ColoSure) for colorectal cancer and pre-cancerous adenomas [9] . Notably, the efficiency of single methylation marker detection is limited not only because multiple pathways and processes are simultaneously altered in tumour cells, but also because colon cancers commonly exhibit different types, evolution, progression and malignancy. Cumulative detection of genetic diseases and tumours at protein, DNA and RNA levels has been demonstrated to be capable of improving detection efficiency [10] , [11] . However, the degree and contribution of promoter methylation in different candidate genes has been rarely taken into account in previous cumulative detection. In recent years, water-soluble cationic conjugated polymers (CCP) have attracted much attention in highly sensitive biosensor applications [12] , [13] . CCPs are highly fluorescent in aqueous media and can amplify the fluorescence intensity of a tightly bound acceptor fluorophore by approximately one order of magnitude through an effective energy transfer pathway [14] . By virtue of the electrostatic interaction between CCP and DNA, extensive optical amplification examples have been demonstrated [15] . Recently, our group has established a simple and highly efficient CCP-based fluorescence resonance energy transfer (FRET) method for analysing gene promoter methylation levels of cancer cells [16] . Compared with the typical PCR-assisted methods, such as Hpa II–PCR [17] , methylation-specific PCR [18] , Ms-SnuPE [19] , COBRA [20] and bisulphite sequencing [21] , our CCP-based FRET method exhibits several advantages. For example, it does not require primer labelling, isolation and washing steps, and is also independent of complicated instruments. Most importantly, our method is suitable for application at the population level because of its sensitivity, simple procedure and label-free characteristics [15] , [16] . In this paper we established the cumulative methylation alteration panels of multiplex genes using the CCP-based methods, and stepwise discriminant analysis on the basis of the methylation levels of a set of candidate genes in tumour tissues and non-cancerous samples. The selected genes contained VIM (GenBank accession number NM_003380 ), adenomatosis polyposis coli ( APC ; GenBank accession number NM_001127511 ), oestrogen receptor 1 ( ESR1 ; GenBank accession number NM_000125 ), mutL homologue 1 ( MLH1 ; GenBank accession number NM_000249 ), transmembrane protein with epidermal growth factor-like and two follistatin-like domains 2 ( TMEFF2/HPP1 ; GenBank accession number NM_016192 ), cyclin-dependent kinase inhibitor 2A ( CDKN2A/P16 ; GenBank accession number NM_058195 ) and O -6-methylguanine–DNA methyltransferase ( MGMT ; GenBank accession number NM_002412 ). It is reported that the aberrant methylation of these genes possesses remarkable significance in the pathogenesis of colon cancer [1] , [3] , [5] , [7] , [22] , [23] , [24] , [25] , [26] , [27] , [28] , [29] , [30] , [31] . Silencing of genes by promoter methylation can inhibit expression of suppressor genes and DNA mismatch repair genes, and cause activation of cancer-related signalling pathway, which underlie the molecular changes in the formation and development of tumours. In addition, the promoters of three CpG island methylator phenotype (CIMP)-related genes, CRABP1 (GenBank accession number: NM_004378 ), NEUROG1 (GenBank accession number: NM_006161 ) and CACNA1G (GenBank accession number: NM_001256327 ) were selected and measured to perform the clinical correlation analysis. In this study, our primary objective is to identify the most promising epigenetic marker combinations out of candidate genes and to establish an efficient discriminant mode for the detection and differential diagnosis of colon cancer. The cumulative detection mode of DNA methylation alterations by CCP-based FRET technique has shown higher accuracy and increased sensitivity in detection and differential diagnosis of colon cancer, suggesting an excellent potential in the clinic applications. CCP-based FRET technique Our paper provided a detailed analysis of methylation degree of colon cancer-related genes using our CCP-based FRET technique [16] . 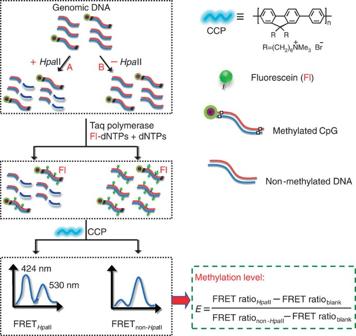Figure 1: Schematic illustration of the CCP-based FRET technique for DNA methylation detection. Methylation protects DNA fromHpaII digestion.HpaII-treated and -untreated DNAs are amplified by PCR in the presence of fluorescein-labelled dNTPs (Fl-dNTPs) followed by adding CCP to allow FRET occurrence when PCR products exist. The methylation level (E) of DNA is calculated according to FRET ratios (I530 nm/I424 nm) ofHpaII-treated, -untreated and blank control samples. Figure 1 depicts the principle of methylation assay using the CCP-based FRET technique. First, the genomic DNAs are extracted from tumour tissues and then digested with restriction endonuclease Hpa II that can recognize the CCGG site and digest the non-methylated DNA, whereas keeping the methylated ones unaffected ( Fig. 1a ). Second, regular PCR is performed to amplify the promoter region. In this step, fluorescein-labelled dNTPs (Fl-dNTPs) are incorporated into the PCR amplicons only for methylated DNAs. Finally, CCP is added into the solution and gives rise to a FRET signal from CCP to fluorescein due to strong electrostatic interactions; in contrast PCR amplification to incorporate Fl-dNTPs into the DNA does not occur for unmethylated DNAs, which does not produce FRET signal. Therefore, the FRET signal for the case of Fig. 1a only originates from the methylated genomic DNAs. For the case in Fig. 1b , genomic DNAs are not treated with Hpa II; thus, regular PCR amplification can incorporate Fl-dNTPs into the amplicons for both methylated and unmethylated DNAs. In this case, the addition of CCP can result in highly efficient FRET signals due to the contribution of the whole genomic DNAs. Given that the relatively quantitative nature is essential to assay the methylation level, herein, parameter E is defined for viewing methylation level with subtracted background by using the equation as shown in Fig. 1 , where the FRET ratio Hpa II refers to the FRET ratio ( I 530 nm / I 424 nm ) for the Hpa II-treated sample, FRET ratio non- Hpa II denotes the FRET ratio for the Hpa II-untreated sample and FRET ratio blank refers to the FRET ratio for the negative non-template control. A high E -value that approaches 1.0 presents a high methylation level, a low E -value that approaches zero presents unmethylation and a mid-value of E presents partial methylation. With the E -value, a standard curve could be plotted versus a series of DNA samples with known methylation content (from 0 to 100%) for calculating the degrees of promoter for clinical samples ( Supplementary Fig. S1 ). Then, by conventional bisulphite sequencing the results of the CCP-based FRET method were validated for part of samples ( Supplementary Table S1 ). Because of the incomplete digestion of restriction enzyme Hpa II and the conditions of PCR amplification, the methylation level detected by the CCP-based FRET method is not absolutely quantitative, and the evaluation for methylation degrees was considered to be semi-quantitative. In addition, the results of detection, differential diagnosis and correlation analysis validate the efficiency of the CCP-based FRET method in practical application. Figure 1: Schematic illustration of the CCP-based FRET technique for DNA methylation detection. Methylation protects DNA from Hpa II digestion. Hpa II-treated and -untreated DNAs are amplified by PCR in the presence of fluorescein-labelled dNTPs (Fl-dNTPs) followed by adding CCP to allow FRET occurrence when PCR products exist. The methylation level ( E ) of DNA is calculated according to FRET ratios ( I 530 nm / I 424 nm ) of Hpa II-treated, -untreated and blank control samples. Full size image To evaluate the efficiency of the CCP-based FRET technique, we tested a known hypermethylated gene promoter of VIM that has been commercially utilized for colon cancer screening [4] . In this experiment, the hypermethylated status was detected for the VIM gene CpG region in 50 normal, 30 colon carcinoma and 30 adenoma cases. As expected, the results show that the medians and averages of methylation levels of VIM in colon carcinoma and adenoma cases are obviously higher than that of the normal control ( P <0.001) in Mann–Whitney’s test ( Fig. 2 ). In view of high efficiency, simple procedure and low cost of the CCP-based FRET technique, several candidate genes were subjected to the methylation analysis in clinical samples. 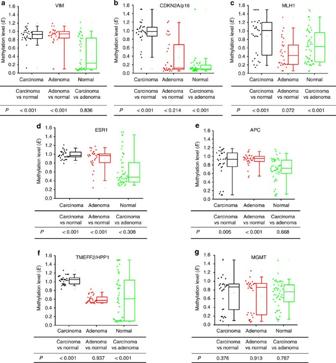Figure 2: Promoter methylation of colon cancer-related genes. (a–g) Box plot representation of methylation detection obtained from seven colon-related genes in 50 normal, 30 colon carcinoma and 30 adenoma cases by using CCP-based FRET technique. Left scatter plots indicate the methylation levels of tested cases. Right plots depict the six-number summaries, namely the minimum and maximum values, the upper (Q3) and lower (Q1) quartiles, median and average values. The median is identified by a line inside the box. The length of the box represents the interquartile range (IQR). Values more than 1.5 IQRs from either end of the box are denoted by an asterisk (*). The square (□) signifies the average. TheP-value is calculated by Mann–Whitney’s test. Figure 2: Promoter methylation of colon cancer-related genes. ( a – g ) Box plot representation of methylation detection obtained from seven colon-related genes in 50 normal, 30 colon carcinoma and 30 adenoma cases by using CCP-based FRET technique. Left scatter plots indicate the methylation levels of tested cases. Right plots depict the six-number summaries, namely the minimum and maximum values, the upper (Q3) and lower (Q1) quartiles, median and average values. The median is identified by a line inside the box. The length of the box represents the interquartile range (IQR). Values more than 1.5 IQRs from either end of the box are denoted by an asterisk (*). The square (□) signifies the average. The P -value is calculated by Mann–Whitney’s test. Full size image Methylation assays of colon cancer-related promoter genes We further employed the CCP-based FRET technique to determine the DNA methylation levels of other six selected gene promoters (CDKN2A/P16, MLH1, ESR1, APC, TMEFF2/HPP1 and MGMT) in 50 normal samples, 30 colon carcinoma and 30 adenoma cases. As shown in Fig. 2 , methylation levels of all gene promoters but MGMT in patients with colon carcinoma are significantly higher than those of the normal control ( P =0.005 or P <0.001, Mann–Whitney’s test), whereas in adenoma cases only the promoters of VIM, ESR1 and APC are more obviously methylated than normal control ( P <0.001, Mann–Whitney’s test). By contrast, no significant difference in methylation levels between the patients and normal population was observed for MGMT ( P >0.05, Mann–Whitney’s test). These results indicate that the methylation level of specific gene promoter associates with different stages of tumour development. Detecting colon cancer by cumulative methylation alteration We hypothesized that a combination of cumulative methylation alterations of multiplexed gene promoters probably increase detection sensitivity. The statistical tools will generate the ideal combination of gene methylation alterations to give the highest possible diagnostic sensitivity and specificity. In this regard, the discriminant analysis was conducted to provide accurate screening information. For the methylation levels of colon cancer-related genes, we employed a detailed Mann–Whitney test to estimate the significance of each of the seven gene promoters in 20 carcinoma and 20 adenoma cases compared with 40 normal controls in terms of P- values ( Supplementary Table S2 ). Consequently, VIM , CDKN2A/P16 , ESR1 and APC genes were preselected for the discriminant analysis and generation of discriminant equations. Through the Wilks’ λ -test in a stepwise method, three out of four genes, VIM, APC and CDKN2A/P16 entered the final mode of the detection. Three co-efficients with discriminant function and one constant construct the discriminant equations that could be used to classify cases. The discriminant equations are shown below: where E is the methylation level value and D is the discriminating value. If D 1 > D 2 , the case belongs to the carcinoma group and vice versa . The classification results based on the D 1 and D 2 values are shown in Table 1 , which clearly shows that 86.3% of original grouped cases are correctly classified with 87.5% sensitivity and 85% specificity in the 40 patients and 40 normal cases. We also validated the detection system and discriminant mode in patients (10 carcinoma and 10 adenoma cases) and 10 normal controls, and 80% of cases ( n =30) could be correctly classified in the validation study ( Supplementary Table S3 ). Table 1 Detection of colon carcinoma or adenoma on the basis of three methylation alterations. * † Full size table Furthermore, we compared the sensitivity of the cumulative methylation detection with that of a single gene detection. The specificity and sensitivity are calculated according to the methylation levels ( E -value) of total 110 samples. As listed in Table 2 , the sensitivity of single gene detection is 51.7% for VIM , 41.7% for APC and 65% for CDKN2A/P16 , respectively, whereas a sensitivity of 86.7% is acquired by using the combination detection mode. These results show that the sensitivity of cumulative mode is significantly enhanced in comparison with that of single detection mode ( P =0.006 or <0.001; χ 2 -test). Table 2 Comparison analysis of combination and single biomarker detection in total 110 samples. Full size table Discrimination between colon carcinoma and adenoma In the present study we found that the methylation levels of CDKN2A/P16, MLH1 and TMEFF2/HPP1 in adenoma cases were significantly different from those of the carcinoma cases, ( P ≤0.001; Mann–Whitney’s test; Supplementary Table S2 ). In contrast, there are no significant differences in methylation levels of other four gene promoters for patients with colon carcinoma and adenoma ( P >0.05; Mann–Whitney’s test). Therefore, CDKN2A/P16, MLH1 and TMEFF2/HPP1 were finally selected to perform discriminant analysis and create the equations. Through the Wilks’ λ -test in a stepwise method, two out of the three genes, TMEFF2/HPP1 and CDKN2A/P16 entered the final mode of the detection. The following equations were achieved: As shown in Table 3 , we analysed 40 known samples and gave a correct classification specificity of 97.5%. Furthermore, the methylation level-based discriminant method was validated and the result shows that all the 20 blind cases, but one, are consistent with that of histological diagnosis ( Supplementary Table S4 ). Table 3 Discrimination of colon carcinoma from adenoma cases on the basis of two combined methylation alterations. * † Full size table Furthermore, we compared the sensitivity of the cumulative methylation detection with that of single gene detection in 50 carcinoma and 50 adenoma cases. As listed in Supplementary Table S5 , the sensitivity of single gene detection is 80% for TMEFF2/HPP1 and 22% for CDKN2A/P16 , respectively, whereas a sensitivity of 94% is acquired by using the combination detection mode. These results show that the sensitivity of cumulative mode is significantly enhanced in comparison with that of the single detection mode ( P =0.0373 and <0.001, respectively; χ 2 -test). CIMP status analysis The methylation levels from the CCP-based FRET were utilized to analyse the relationship between CIMP status and clinical characteristics. Fifty carcinoma cases were divided into CIMP-high (H), -low (L) and –negative (N) groups according to the methylation status of the nine gene promoters. The markers of the CIMP panel include VIM, TMEFF2/HPP1, CDKN2A/p16, MLH1, ESR1 and APC, which were significantly methylated in the CpG islands in the carcinoma cases compared with normal controls ( Fig. 1 ). To accurately classify the CIMP, three well-known CIMP markers were also chosen and measured by the CCP-based FRET method. Clinical characteristics of the patients are summarized in Supplementary Table S6 . In this study, between the CIMP N, CIMP L and CIMP H groups there were no significant differences in sex and age ( P >0.05). However, the frequency of the case of serosa invasion was significantly higher in the CIMP H group (68.2%; P =0.009, χ 2 -test) than in the CIMP N and CIMP L groups. In addition, the cases of the CIMP H group was more common in the poor differentiation tumours (45.5%) than other groups (≤ 20.0%; Table 4 ). More proximal tumours exhibited a CIMP H status ( Supplementary Table S10 ).Our findings showed that the CIMP status appeared to be correlated with tumour progression and cell differentiation degree. Table 4 Correlation analysis of CIMP status and clinical parameter in 50 carcinomas cases Full size table We have performed a cumulative analysis of multiple methylated genes to detect and differentiate colon cancer by using the CCP-based FRET technique and discriminant analysis. Compared with conventional methods, the unique features of our method are its high efficiency, simple procedure and low cost [15] . In addition, this method provides a semi-quantitative analysis of differential DNA methylation levels. The results from known hypermethylated gene ( VIM ) demonstrate that both adenoma and carcinoma groups exhibit significant promoter methylation levels in comparison with normal control ( Fig. 1 ), which is consistent with previous research findings [7] , [8] . Results from other six genes are also in substantial agreement with those in the literatures [5] , [28] . For instance, consistent with the results of the studies of Goto et al . [23] , Petko et al . [24] and Kane et al . [25] , CDKN2A/p16 and MLH1 are significantly or aberrantly methylated in colon carcinoma or advanced adenomas cases. Noted that some results show contrary conclusions to some reported results, Lee et al . [26] and Bariol et al . [27] found there was no significant difference in the frequencies of CDKN2A/p16 and MGMT methylations between the colon adenoma and cancer. We could not detect increased methylation levels of MGMT in the 60 patients compared with the 50 normal controls ( Fig. 1 ). There are multiple potential reasons for the difference including assay-related differences, environmental factors and differing patient populations. Despite the contradictory results to several reports, the obvious differences of methylation levels in all the selected genes, but MGMT , were observed between the carcinoma/adenoma cases and normal controls by employing the CCP-based FRET technique ( Fig. 1 ). The above results demonstrate that our data could truly represent the promoter methylation status of the tested genes. Most importantly, the present study has demonstrated a new cumulative detection mode. In our experiments, two sets of discriminant equations were deduced by stepwise discriminant statistical method, and after having utilized the two sets of equations we took into account the role of multiple methylation alterations in the tumour development and progression. We detected and analysed the aberrantly methylated genes in the adenoma and carcinoma tissues, and found that most patients carried at least one methylated allele within the VIM, APC, ESR1, MLH1, TMEFF2/HPP1 and CDKN2A/P16. Notably, the methylation levels of VIM, CDKN2A/p16, APC and TMEFF2/HPP1 are significantly higher in the adenoma and carcinoma cases than those of the controls ( Fig. 1 and Supplementary Table S2 ). Through the discriminant analysis, three highly related genes enter the final discriminant equations (1) and (2). According to methylation levels of the 110 tested samples, the cumulative detection can reach a sensitivity of 86.7%, whereas only 41.7–65% detection sensitivity was obtained by single methylation detection mode ( Table 2 ). It is noted that for VIM methylation screening based on methylation detection of single gene, a similar sensitivity of 46% and specificity of 90% were achieved by the study of Chen et al .’s [8] group. Therefore, by using the CCP-based FRET technique, cumulative detection for multiple genes of promoters can increase the detection efficiency. It should be noted this technique exhibits high detection sensitivity so that little DNA samples obtained from serum, plasma or stool can be used for methylation analysis. So, it would be a useful tool for early screening in variously derived DNA samples, including tumour tissues, as a non-invasive mode. Besides the screening of colon cancer, our new technique can also perform differential diagnosis. Most colon cancers may begin as an adenoma that evolves into carcinoma, and specific gene methylation occurs in CpG regions of promoter during malignant transformation. Our data reveal that some gene methylations occur at the early tumour stages and the methylation contributes to later stages of colon carcinogenesis, whereas some gene methylations cannot be observed until the later stages ( Fig. 1 ). Accurately classifying histological types will be essential to perform anti-cancer therapy and assess prognosis. Through the stepwise discriminant analysis, CDKN2A/P16 and TMEFF2/HPP1 were used to construct the discriminant equations (3) and (4). These results demonstrate a high efficiency, except for one false sample in the 40 test samples and 20 blind ones, which indicates that the cumulative detection of stage-specific methylation biomarkers could complement and confirm the histological diagnosis results. In addition, with the data of methylation degree obtained using the CCP-based FRET method, we could evaluate the correlation between methylation status and clinical parameters. In this study, we employed a panel of nine CIMP markers to analyse the relationship. Our data demonstrate that CIMP H status is significantly correlated with the deep invasion in this study. The results of correlation analysis are in agreement with the Hinoue et al . [29] and Dahlin et al .’s [30] reports that more proximal tumours were observed in the CIMP H group when compared with the CIMP L or N groups [29] , [30] , [31] . CIMP N tumours more often have well and moderate degree of tumour differentiation, although there are not statistical significant differences between the groups. Dahlin et al .’s [30] group also reported the similar findings in microsatellite instability (MSI) patients. Because of different populations, limited sample number, CIMP markers, technical approaches, MSI, gene mutation status and so on, our results are partially not consisted with previous reports [31] , [32] ; however, the semi-quantitative CCP-based FRET method supplies a robust tool for identifying the significance of multiple CIMP panel markers in tumour development. More recently, a novel colorectal continuum theory was proposed and confirmed based on the analysing molecular features of 1,443 colorectal cancers. The findings by Yamauchi [33] showed that the molecular features (CIMP H, MSI H and BRAF mutations) might gradually change along bowel subsites, rather than change abruptly at splenic flexure. Because of the limited number and types of tumour samples, we can only preliminarily analyse the relation between the CIMP status and tumour location according to the typical classification standard ( Supplementary Table S10 ). Notably, to extend the application of the CCP-based FRET technology in the fields of clinical, translational and epidemiology research, a large-scale cancer database needs to be comprehensively investigated further. Besides the accumulated genetic and epigenetic alterations in cancer cells, there has been increasing interest in the tumour microenvironment. For example, cancer-assisting proteins in the stromal tissue might be one of mechanisms of drug resistance [34] . The bacteria and viruses can also directly or indirectly mediate cancer development [35] . All the factors can result in cancer transformation and development by various genetic and epigenetic alterations and other specific mechanisms. In summary, we analysed semi-quantitatively the DNA methylation levels of seven critical genes in patients with colon carcinoma, adenoma and in healthy controls in a Chinese population. Through a stepwise discriminant analysis and cumulative methylation alterations, a correct classification rate of 86.3% was obtained for patients with colon adenoma and pre-cancerous carcinoma. Meanwhile, carcinoma cases could be distinguished from adenoma cases with an accuracy of 97.5%. Compared with the single methylation biomarker detection, the newly developed cumulative detection mode also results in a higher sensitivity. Moreover, the CCP-based FRET method could also be used in clinical correlation analysis. Although the number of samples in the present study is limited, our findings have shown that the combination of three genes can be used to discriminate carcinoma/adenoma and normal case, and the combination of two genes can be used to discriminate adenoma from carcinoma. Thus, a cumulative detection of highly colon cancer-related gene methylation alterations will open a new field for early detection and differential diagnosis by using our CCP-based FRET technique and discriminant analysis in a cheap, simple and non-invasive mode. These epigenetic biomarker detections can also predict the clinical outcome of methylation inhibitor-based chemotherapy [36] . Tissue samples and DNA extraction To establish and validate a discrimination mode for detection and differential diagnosis of colon cancer, we retrospectively studied 30 colon carcinoma and 30 adenoma patients (48% men, 52% women and aged from 31 to 85 years). To evaluate the sensitivity, the differential diagnosis using the mode and the relationship between the clinical parameters and CIMP status, additional 20 colon carcinoma and 20 adenoma samples were also detected using the CCP-based FRET method. These cases underwent surgery between August 2003 and January 2004, and gave written informed consent for DNA isolation and employment. The study was approved by the local institutional review board. We also isolated DNA from 50 healthy people as the control group. The normal controls were non-carcinoma, non-adenoma and non-inflammatory samples. The 50 carcinoma patients’ characteristics were included in detail in Supplementary Table S5 . To decrease the fraction of normal tissue contamination in collected samples, the sections stained with haematoxylin-eosin staining were reviewed and re-examined by the same pathologist. Genomic DNAs of formalin-fixed and paraffin-embedded tissue sections were isolated and extracted with QIAamp DNA blood mini kit (QIAGEN). Briefly, the tissue samples were lysed thoroughly with lysis buffer containing proteinase K, followed by incubating at 56 °C for 10 min or overnight, and equal volume of 100% ethanol were then added. After passing through the QIAamp spin mini column, the genomic DNAs bound to the column. Pure genomic DNAs were collected by washing twice and then eluting. To extract the DNA from formalin-fixed and paraffin-embedded tissues, eight 10-μm thick sections were cut from the samples and cleared of paraffin by treatment with xylene, and then rinsed with 100% ethanol. Because of different amounts and possible degradation of DNA during the preparation procedure, we checked all samples for their DNA contents. DNA concentration and quality were evaluated by absorbance at 260 and 280 nm using Nanodrop Spectrophotometers (Thermo Scientific, ND2000), respectively. Gene selection for methylation analysis We selected several colon cancer-related genes based on the findings in the published literatures. They are associated with transcriptional silencing of various genes including tumour suppressor genes and genes involved in DNA repair and apoptosis. Seven genes were selected to determine the methylation levels of their promoters that could be most promising epigenetic markers to identify patients with colon cancer. These tested genes include VIM , APC , ESR1 , MLH1 , TMEFF2/HPP1 , CDKN2A/P16 and MGMT . All the gene sequences are available at online website, http://:www.ensembl.org . Detection of promoter methylation level For detecting the methylation status, seven genes containing promoter regions were amplified by PCR. All the amplicons cover at least two CCGG sites and the primer sequences are listed in Supplementary Table S7 . Then, DNA methylation level was detected by using the CCP-based FRET method [17] . Briefly, genomic DNA was digested with HpaII (New England Biolabs) at 37 °C for 24 h. The reaction system comprised 200 ng of genomic DNA, 20 U of HpaII (New England Biolabs), 2 μl of 10 × Hpa II buffer I and sterile H 2 O. The resulted DNA was used for PCR amplification or stored at −80 °C. Then, the Hpa II-digested DNA was PCR amplified and the PCR conditions were as follows: 95 °C for 4 min, followed by 40 cycles at 95 °C for 30 s and 60 °C for 30 s, 72 °C for 40 s, and a final extension at 72 °C for 10 min. For incorporating the Fl-dNTPs, the second PCR was performed by using the first round PCR products as templates. The methylation levels were calculated by the equation (5) as shown below: where FRET ratio Hpa II refers to FRET ratio ( I 530 nm / I 424 nm ) for the Hpa II-treated sample, FRET ratio non- Hpa II denotes the FRET ratio for the Hpa II-untreated sample and FRET ratio blank refers to the FRET ratio for the negative non-template control. The fully methylated and unmethylated DNA samples confirmed by the bisulphite sequencing were mixed with the methylation percentages from 0, 0.79, 1.59, 3.18, 6.25, 12.5, 25, 50 and 75 up to 100%. With the E -value obtained using the CCP-based FRET method, a standard curve was plotted versus the series of DNA samples with the known methylation degree (from 0 to 100%). To confirm the semi-quantitative results obtained from the CCP-based FRET method, the methylation levels of CpG islands in part of samples were detected using the bisulphite sequencing. The bisulphite sequencing experiment was described in the section of Supplementary Methods . CIMP status analysis To analyse the relationship between the CIMP status and various clinical parameters, three additional CIMP-related genes, CRABP1 , NEUROG1 and CACNA1G were detected using the CCP-based FRET method. The PCR primers are listed in Supplementary Table S8 . Besides three well-known genes for CIMP classification, the CIMP panel consists of CpG islands from the following genes: VIM , TMEFF2 / HPP1 , CDKN2A / p16 , MLH1 , ESR1 and APC . For each carcinoma sample, E -values of methylation levels more than the value of 80% normal samples were defined as positive samples. In this analysis, the CIMP H was defined as the presence of five or more methylated promoters among the nine markers; the CIMP L was defined as one to four methylated promoters; and the CIMP N was defined as the absence of methylated promoters. Statistical analysis Statistical analysis of methylation data was performed using the SPSS 17.0 software. The differences of each gene methylation alteration between two groups were tested with the Mann–Whitney’s test. The χ 2 -test was used to compare the sensitivity of combination detection versus single methylation alteration detection. The relations between the CIMP status and clinical parameters were also tested with one-way analysis of variance, χ 2 -test or Fisher’s exact test. Differences were considered to be significant for P <0.05. The preselected genes with significant difference by Mann–Whitney’s test were included in the discriminant analysis to detect carcinoma and adenoma cases from the normal and to distinguish carcinoma and adenoma. In the discriminant analysis, we selected the stepwise discrimination analysis using the Wilk’s λ -criterion. To confirm the discriminant modes, two sets of validation studies were carried out. The methylation levels of selected genes from each sample were used in the discriminant equations to determine their status (colon carcinoma/adenoma or normal). How to cite this article: Yang, Q. et al . Detection and differential diagnosis of colon cancer by a cumulative analysis of promoter methylation. Nat. Commun. 3:1206 doi: 10.1038/ncomms2209 (2012).